Tricritical wings and modulated magnetic phases in LaCrGe3under pressure 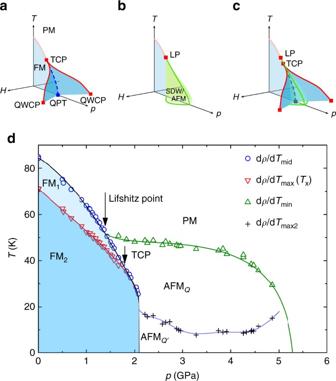Fig. 1 Temperature–pressure phase diagram.aSchematicT-p-Hphase diagram of a quantum ferromagnet: the paramagnetic-ferromagnetic (PM-FM) transition becomes of the first order at a tricritical point (TCP) after which there is a quantum phase transition (QPT) at 0 K. Tricritical wings emerge from the TCP under magnetic field and terminate at quantum wing critical points (QWCP).bSchematicT-p-Hphase diagram of a quantum ferromagnet when a modulated magnetic phase (SDW/AFM) emerges from the Lifshitz point (LP).cNew possible schematicT-p-Hphase diagram for which tricritical wings as well as a new magnetic phase are observed.dT-pphase diagram of LaCrGe3from electrical resistivity measurements16showing two FM regions (FM1 and FM2) separated by a crossover. Thesolid linesare guides to the eye Experimental and theoretical investigations on itinerant ferromagnetic systems under pressure have shown that ferromagnetic quantum criticality is avoided either by a change of the transition order, becoming of the first order at a tricritical point, or by the appearance of modulated magnetic phases. In the first case, the application of a magnetic field reveals a wing-structure phase diagram as seen in itinerant ferromagnets such as ZrZn 2 and UGe 2 . In the second case, no tricritical wings have been observed so far. Here, we report on the discovery of wing-structure as well as the appearance of modulated magnetic phases in the temperature-pressure-magnetic field phase diagram of LaCrGe 3 . Our investigation of LaCrGe 3 reveals a double-wing structure indicating strong similarities with ZrZn 2 and UGe 2 . But, unlike these simpler systems, LaCrGe 3 also shows modulated magnetic phases similar to CeRuPO. This finding provides an example of an additional possibility for the phase diagram of metallic quantum ferromagnets. Suppressing a second-order, magnetic phase transition to zero temperature with a tuning parameter (pressure, chemical substitutions, magnetic field) has been a very fruitful way to discover many fascinating phenomena in condensed matter physics. In the region near the putative quantum critical point (QCP), superconductivity has been observed in antiferromagnetic [1] as well as ferromagnetic (FM) systems [2] , [3] , [4] . One peculiarity of the clean FM systems studied so far is that the nature of the paramagnetic-ferromagnetic (PM-FM) phase transition always changes before being suppressed to zero temperature [5] : in most cases, the transition becomes of the first order [6] , [7] , [8] , [9] , [10] , [11] . Recently, another possibility, where a modulated magnetic phase (AFM Q ) appears (spin-density wave, antiferromagnetic order), has been observed in CeRuPO [12] , [13] , MnP [14] , [15] , and LaCrGe 3 [16] . Several theories have been developed to explain those possibilities [17] , [18] , [19] , [20] , [21] , [22] , [23] , [24] , [25] , [26] . When a FM transition becomes of the first order at a tricritical point (TCP) in the temperature T pressure p plane, the application of a magnetic field H along the magnetization axis reveals a wing structure phase diagram in the T - p - H space [20] , [27] . This is seen in UGe 2 [28] , [29] and ZrZn 2 [30] and is schematically represented in Fig. 1a . This phase diagram shows the possibility of a different kind of quantum criticality at the quantum wing critical point (QWCP). In contrast with the conventional QCP, symmetry is already broken by the magnetic field at a QWCP. In the more recently considered case where the transition changes to a AFM Q phase, no wing structure phase diagram has been reported, but it is found that the AFM Q is suppressed by moderate magnetic field [12] , [13] . This second possible T - p - H phase diagram has been schematically presented in a recent review [5] and reproduced in Fig. 1b . Fig. 1 Temperature–pressure phase diagram. a Schematic T - p - H phase diagram of a quantum ferromagnet: the paramagnetic-ferromagnetic (PM-FM) transition becomes of the first order at a tricritical point (TCP) after which there is a quantum phase transition (QPT) at 0 K. Tricritical wings emerge from the TCP under magnetic field and terminate at quantum wing critical points (QWCP). b Schematic T - p - H phase diagram of a quantum ferromagnet when a modulated magnetic phase (SDW/AFM) emerges from the Lifshitz point (LP). c New possible schematic T - p - H phase diagram for which tricritical wings as well as a new magnetic phase are observed. d T - p phase diagram of LaCrGe 3 from electrical resistivity measurements [16] showing two FM regions (FM1 and FM2) separated by a crossover. The solid lines are guides to the eye Full size image Here, we report electrical resistivity measurements on LaCrGe 3 under pressure and magnetic field. We determine the T - p - H phase diagram and find that it corresponds to a third possibility where tricritical wings emerge in addition to the AFM Q phase. This type of phase diagram is illustrated in Fig. 1c : it includes both the tricritical wings and the AFM Q phase. In addition, the phase diagram of LaCrGe 3 shows a double wing structure similar to what is observed in the itinerant ferromagnets UGe 2 [31] and ZrZn 2 [32] , but with the additional AFM Q phase. LaCrGe 3 is the first example showing such a phase diagram. T - p phase diagram Recently, we reported on the T - p phase diagram of LaCrGe 3 [16] , which is reproduced in Fig. 1d . At ambient pressure, LaCrGe 3 orders ferromagnetically at TC = 86 K. Under applied pressure, TC decreases and disappears at 2.1 GPa. Near 1.3 GPa, there is a Lifshitz point [33] at which a new transition line appears. The transition corresponds to the appearance of a modulated magnetic phase (AFM Q ) and can be tracked up to 5.2 GPa. Muon-spin rotation (μSR) measurements show that the AFM Q phase has a similar magnetic moment as the FM phase but without net macroscopic magnetization [16] . In addition, band structure calculations suggest that the AFM Q phase is characterized by a small wave-vector Q and that several small Q phases are nearly degenerate. Below the PM-AFM Q transition line, several anomalies marked as gray cross in Fig. 1d can be detected in ρ ( T ) [16] . These other anomalies within the AFM Q phase are compatible with the near degeneracy of different Q -states (shown as AFM Q and AFM Q ′ ) with temperature and pressure driven transitions between states with differing wavevectors. In this article, we determine the three dimensional T - p - H phase diagram of LaCrGe 3 by measuring the electrical resistivity of single crystals of LaCrGe 3 under pressure and magnetic field. FM1 and FM2 phases Whereas most of the features in Fig. 1d were well understood in ref. [16] , we also indicate the pressure dependence of T x (d ρ /d T max ) at which a broad maximum is observed in d ρ/ d T below TC and shown as orange triangles in Fig. 1d . At ambient pressure, T x ≈ 71 K. No corresponding anomaly can be observed in magnetization [16] , internal field [16] or specific heat [34] . Under applied pressure, T x decreases and cannot be distinguished from TC (d ρ /d T mid ) above 1.6 GPa. As will be shown, application of magnetic field allows for a much clearer appreciation and understanding of this feature. 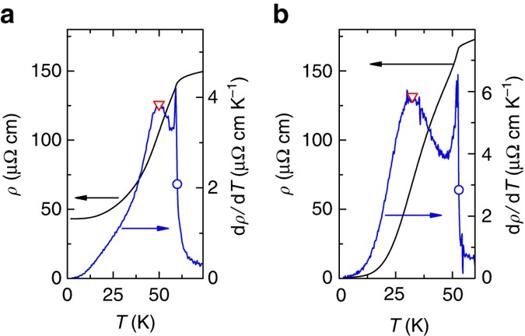Fig. 2 Comparison ofρ(T) and its dρ(T)/dTbetween LaCrGe3and UGe2. Temperature dependence of the resistivity (black line,left axis) and its derivative (blue line,right axis) ofaLaCrGe3at 1.14 GPa andbUGe2at 0 GPa from ref.28. The crossover between the two ferromagnetic phases (FM1 and FM2) is inferred from the maximum in dρ/dT(Tx) and marked by ared triangle, whereas the paramagnetic-ferromagnetic transition is inferred from the middle point of the sharp increase in dρ/dT(TC) and indicated by ablue circle Figure 2a shows the anomalies at T x and T C observed in the electrical resistivity and its temperature derivative at 1.14 GPa. For comparison, Fig. 2b shows ambient pressure data for UGe 2 [28] where a similar anomaly at T x can be observed. In UGe 2 , this anomaly was studied intensively [35] , [36] , [37] . It corresponds to a crossover between two ferromagnetic phases FM1 and FM2 with different values of the saturated magnetic moment [35] , [36] . Under pressure, there is a critical point at which the crossover becomes a first-order transition, which eventually vanishes where a maximum in superconducting-transition temperature is observed [2] . In the case of LaCrGe 3 , we cannot locate where the crossover becomes a first order transition, since the anomaly merges with the Curie temperature anomaly near 1.6 GPa, very close to the TCP. However, as we will show below, the two transitions can be separated again with applied magnetic field above 2.1 GPa. This is similar to what is observed in UGe 2 where the PM-FM1 and FM1-FM2 transition lines separate more and more as the pressure and the magnetic field are increased. Because of such similarities with UGe 2 , we label the two phases FM1 and FM2 and assume that the anomaly at T x corresponds to a FM1-FM2 crossover. A similar crossover was also observed in ZrZn 2 [32] . In refs [18] , [25] , a Stoner model with two peaks in the density of states near the Fermi level was proposed to account for the two phases FM1 and FM2, reinforcing the idea of the itinerant nature of the magnetism in LaCrGe 3 . Fig. 2 Comparison of ρ ( T ) and its d ρ ( T )/d T between LaCrGe 3 and UGe 2 . Temperature dependence of the resistivity ( black line , left axis ) and its derivative ( blue line , right axis ) of a LaCrGe 3 at 1.14 GPa and b UGe 2 at 0 GPa from ref. [28] . The crossover between the two ferromagnetic phases (FM1 and FM2) is inferred from the maximum in d ρ /d T ( T x ) and marked by a red triangle , whereas the paramagnetic-ferromagnetic transition is inferred from the middle point of the sharp increase in d ρ /d T ( TC ) and indicated by a blue circle Full size image Field-dependent resistivity measurement under pressure In zero field, for applied pressures above 2.1 GPa, both FM1 and FM2 phases are suppressed. Upon applying a magnetic field along the c -axis, two sharp drops of the electrical resistivity can be observed (Fig. 3a ) with two corresponding minima in the field derivatives (Fig. 3b ). At 2 K, clear hysteresis of Δ H ~ 0.7 T can be observed for both anomalies indicating the first order nature of the transitions. The emergence of field-induced first-order transitions starting from 2.1 GPa and moving to higher field as the pressure is increased (Supplementary Note 1 ) is characteristic of the FM quantum phase transition: when the PM-FM transition becomes of the first order, a magnetic field applied along the magnetization axis can induce the transition resulting in a wing structure phase diagram such as the one illustrated in Fig. 1a . In the case of LaCrGe 3 , evidence for a first order transition was already pointed out because of the very steep pressure dependence of T C near 2.1 GPa and the abrupt doubling of the residual ( T = 2 K) electrical resistivity [16] . In UGe 2 or ZrZn 2 , the successive metamagnetic transitions correspond to the PM-FM1 and FM1-FM2 transitions. In LaCrGe 3 , at 2 K, due to the presence of the AFM Q ′ phase at zero field, the transitions correspond to AFM Q ′ -FM1 and FM1-FM2. Fig. 3 Determination of wing critical point at 2.39 GPa. a Field dependence of the electrical resistivity at 2, 13.5, and 30 K at 2.39 GPa with applied field along the c -axis. Continuous and dashed lines represent the field increasing and decreasing, respectively. When the continuous and dashed lines do not overlap, there is indication for hysteresis. b Corresponding field derivatives (d ρ /d H ). The curves are shifted by 15 μΩ cm T −1 for clarity. Vertical arrows represent the minima. The transition width is determined by the full width at half minimum as represented by horizontal arrows . Solid and open symbols in a , b represent the transition fields for field increasing and decreasing ( squares for AFM Q -FM1 and circles for FM1-FM2). The blue cross symbols in a , b represent the AFM Q -PM transition at this pressure. The temperature dependence of the hysteresis width of H min1 and H min2 ( solid symbols ) are shown in c , d ( left axes ). The hysteresis width gradually decreases with increasing temperature and disappears at Tw corresponding to the wing critical point ( vertical red arrows ). The right axes show the temperature dependence of the transition widths ( open symbols ). Dashed lines are guides to the eye. The width is small for the first-order transition and becomes broad in the crossover region. The blue-color shaded area represents the first order transition region, whereas the white color area represents the crossover region. These allow for the determination of the wing critical point of the FM1 transition at 13.5 ± 1.5 K, 2.39 GPa, and 5.1 T and the one for the FM2 transition at 12 ± 1 K, 2.39 GPa and 7.7 T Full size image Determination of the wing structure phase diagram As the temperature is increased, the hysteresis decreases for both transitions, as can be seen in Fig. 3c , d and disappears at a wing critical point (WCP). Also, the transition width is small and weakly temperature dependent below the WCP and it broadens when entering in the crossover regime. Similar behavior has been observed in UGe 2 [29] . At 2.39 GPa for example, we locate the WCP of the first-order FM1 transition around 13.5 K and the one of the first-order FM2 transition around 12 K. At this temperature and pressure, the transitions occur at 5.1 and 7.7 T, respectively. This allows for the tracking of the wing boundaries in the T - p - H space up to our field limit of 14 T. At low field, near the TCP, the wing boundaries are more conveniently determined as the location of the largest peak in d ρ /d T (Supplementary Note 2 ). The projections of the wings lines T w ( p , H ) in the T - H , T - p , and H - p planes are shown in Fig. 4a–c, respectively. The metamagnetic transitions to FM1 and FM2 start from 2.1 GPa and separate in the high field region as the pressure is further increased. For the FM1 wing, the slope d T w /d H w is very steep near H = 0 (Fig. 4a ), whereas d H w /d p w is very small (Fig. 4c ). This is in agreement with a recent theoretical analysis based on the Landau expansion of the free energy, which shows that d T w /d H w and d p w /d H w are infinite at the TCP [27] . This fact was overlooked in the previous experimental determinations of the wing structure phase diagram in UGe 2 [28] , [29] and ZrZn 2 [30] , but appears very clearly in the case of LaCrGe 3 . In the low field region, there are no data for the FM2 wing since the transition is not well separated from the FM1 wing, but there is no evidence for an infinite slope near H = 0. The wing lines can be extrapolated to QWCPs at 0 K in high magnetic fields of the order of ~30 T (Fig. 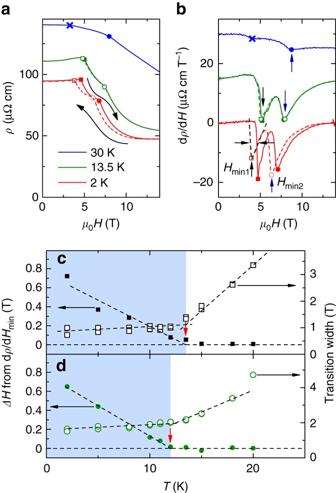Fig. 3 Determination of wing critical point at 2.39 GPa.aField dependence of the electrical resistivity at 2, 13.5, and 30 K at 2.39 GPa with applied field along thec-axis.Continuousanddashed linesrepresent the field increasing and decreasing, respectively. When thecontinuousanddashed linesdo not overlap, there is indication for hysteresis.bCorresponding field derivatives (dρ/dH). The curves are shifted by 15 μΩ cm T−1for clarity.Vertical arrowsrepresent the minima. The transition width is determined by the full width at half minimum as represented byhorizontal arrows.Solidandopen symbolsina,brepresent the transition fields for field increasing and decreasing (squaresfor AFMQ-FM1 andcirclesfor FM1-FM2). Theblue cross symbolsina,brepresent the AFMQ-PM transition at this pressure. The temperature dependence of the hysteresis width ofHmin1andHmin2(solid symbols) are shown inc,d(left axes). The hysteresis width gradually decreases with increasing temperature and disappears atTwcorresponding to the wing critical point (vertical red arrows). Theright axesshow the temperature dependence of the transition widths (open symbols).Dashed linesare guides to the eye. The width is small for the first-order transition and becomes broad in the crossover region. Theblue-colorshaded arearepresents the first order transition region, whereas thewhite colorarearepresents the crossover region. These allow for the determination of the wing critical point of the FM1 transition at 13.5 ± 1.5 K, 2.39 GPa, and 5.1 T and the one for the FM2 transition at 12 ± 1 K, 2.39 GPa and 7.7 T 4a ) and pressures around ~3 GPa (Fig. 4b ). Fig. 4 Shape of the tricritical wing lines ( T w , p w , H w ). Projection of the wings in a T - H , b T - p and c H - p planes. Black solid squares and green solid circles represent the FM1-wing and FM2-wing, respectively. Red lines (represented in the T - p - H space in Fig. 5 ) are guides to the eyes and open symbols represent the extrapolated quantum wing critical point (QWCP). d H - p phase diagram at 2 K. The arrow represents the pressure p c = 2.1 GPa. The green color cross symbols represent the AFM Q ′ phase boundary. Dark blue , light blue , and green color shaded areas represent the FM2, FM1, and AFM Q ′ phases, respectively. The error bars in pressure for b – d are determined by the superconducting transition width of the Pb manometer. 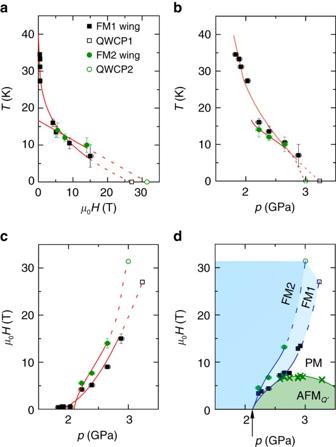Fig. 4 Shape of the tricritical wing lines (Tw,pw,Hw). Projection of the wings inaT-H,bT-pandcH-pplanes.Black solid squaresandgreen solid circlesrepresent the FM1-wing and FM2-wing, respectively.Red lines(represented in theT-p-Hspace in Fig.5) are guides to the eyes andopen symbolsrepresent the extrapolated quantum wing critical point (QWCP).dH-pphase diagram at 2 K. Thearrowrepresents the pressurepc= 2.1 GPa. Thegreen colorcross symbolsrepresent the AFMQ′phase boundary.Dark blue,light blue, andgreen colorshaded areasrepresent the FM2, FM1, and AFMQ′phases, respectively. Theerror barsin pressure forb–dare determined by the superconducting transition width of the Pb manometer. Fora–d, theerror barsin temperature and magnetic field are determined as half the data spacing 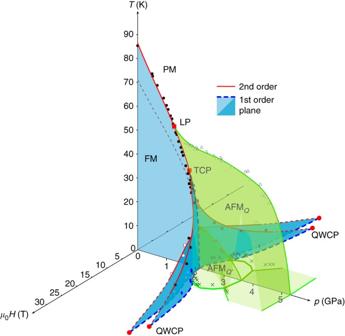Fig. 5 T-p-Hphase diagram of LaCrGe3.Red solid linesare the second order phase transition andblue colorplanesare planes of first order transitions.Green colorareasrepresent the AFMQand AFMQ′phases. For clarity, only data points at 2 K and along the transitions lines are shown.Black circlesindicate the paramagnetic (PM)-ferromagnetic (FM) transition.Black squaresindicate the wing critical line for FM1 andempty squaresindicate the wing critical line for FM2.Blue diamondsindicate the first order transition to the FM1 state at 2 K andempty diamonds, the first order transition to FM2 at 2 K.Empty trianglesindicate the PM-modulated magnetic phase (AFMQ) and “+” indicate the AFMQ′boundary. “×” indicate the AFMQor AFMQ′boundary at 2 K. The full set of data points can be found in Supplementary Note3. For clarity, thegreen surfacesrepresenting the boundaries for the AFMQor AFMQ′phases are shown only in the region of positive magnetic field For a – d , the error bars in temperature and magnetic field are determined as half the data spacing Full size image Figure 4d shows the H - p phase diagram at low temperature ( T = 2 K). The magnetic field at the transition to the FM1 phase increases rapidly, whereas the field suppressing the AFM Q ′ phase does not exceed 7 T. Above 2.5 GPa, the AFM Q ′ and FM1 phases are separated by a region corresponding to the polarized PM phase. We note that a similar diagram where the wings extend beyond the AFM phase was recently obtained theoretically in the case of strong quantum fluctuations effects [38] . The similarity of the H - p phase diagram at 2 K (Fig. 4d ) and the projection of the wings in the H - p plane (Fig. 4c ) reveals the near vertical nature of the wings. T-p-H phase diagram of LaCrGe 3 The resulting three-dimensional T - p - H phase diagram of LaCrGe 3 is shown in Fig. 5, which summarizes our results (Several of the constituent T - H phase diagrams, at various pressures, are given in Supplementary Fig. 3 ). The double wing structure is observed in addition to the AFM Q phase. This is the first time that such a phase diagram is reported. Other materials suggested that there is either a wing structure without any additional magnetic phase [28] , [29] , [30] , or a magnetic phase without a wing structure [12] , [13] . The present study illustrates a third possibility where all such features are observed. The phase diagram of LaCrGe 3 and the existence of wings clearly establish that the quantum phase transition from FM to AFM Q ′ is of the first order. It is plausible that the reason is the same as for the FM to PM transition, but no theory is available for this case, as pointed out in a recent review [5] . Another interesting aspect is the existence of the two metamagnetic transitions (to FM1 and FM2) which suggests that this might be a generic feature of itinerant ferromagnetism. Indeed, it is observed in ZrZn 2 , UGe 2 , and LaCrGe 3 , although these are very different materials with different electronic orbitals giving rise the the magnetic states. We note that a wing structure has also been determined in the PM compounds UCoAl [39] , [40] , [41] and Sr 3 Ru 2 O 7 [42] , implying that a FM state probably exists at negative pressures in these materials. Strikingly, two anomalies could be detected upon crossing the wings in UCoAl (two kinks of a plateau in electrical resistivity [39] , two peaks in the ac susceptibility [41] ), as well as in Sr 3 Ru 2 O 7 (two peaks in the ac susceptibility [42] ). These double features could also correspond to a double wing structure. Fig. 5 T - p - H phase diagram of LaCrGe 3 . Red solid lines are the second order phase transition and blue color planes are planes of first order transitions. Green color areas represent the AFM Q and AFM Q ′ phases. For clarity, only data points at 2 K and along the transitions lines are shown. Black circles indicate the paramagnetic (PM)-ferromagnetic (FM) transition. Black squares indicate the wing critical line for FM1 and empty squares indicate the wing critical line for FM2. Blue diamonds indicate the first order transition to the FM1 state at 2 K and empty diamonds , the first order transition to FM2 at 2 K. Empty triangles indicate the PM-modulated magnetic phase (AFM Q ) and “+” indicate the AFM Q ′ boundary. “ × ” indicate the AFM Q or AFM Q ′ boundary at 2 K. The full set of data points can be found in Supplementary Note 3 . For clarity, the green surfaces representing the boundaries for the AFM Q or AFM Q ′ phases are shown only in the region of positive magnetic field Full size image Conclusions To conclude, the T - p - H phase diagram of LaCrGe 3 provides a distinct example of possible outcomes of FM quantum criticality. At zero field, quantum criticality is avoided by the appearance of a new modulated magnetic phase, but the application of magnetic field shows the existence of a wing structure phase diagram leading towards QWCP at high field. These experimental findings reveal insights into the possible phase-diagrams of FM systems. The emergence of the wings reveals a theoretically predicted tangent slope [27] near the TCP, a fact that was overlooked in previous experimental determination of phase diagrams of other compounds because of the lack of data density in that region. In addition, the double nature of the wings appears to be a generic feature of itinerant ferromagnetism, as it is observed in several, a priori, unrelated materials. This result deserves further theoretical investigations and unification. Sample preparation Single crystals of LaCrGe 3 were grown using a high-temperature solution growth technique [43] , [44] . A mixture of La, Cr, and Ge with a molar ratio of La:Cr:Ge = 13:13:74 was premixed by arc melting. The material was then placed in a 2-mL alumina crucible and sealed in a silica ampoule under partial pressure of high purity argon gas. The sealed ampoule was heated to 1100 °C over 3 h and held for 5 h. After that, it was cooled to 825 °C and the remaining liquid was decanted using a centrifuge. Details about the crystal growth procedure and sample characterization at ambient pressure is described in ref. [34] . The resistivity measurements under pressure The samples for the pressure study were selected after ambient pressure characterization by the magnetization and resistivity measurements. Temperature and field dependent resistance measurements were carried out using a Quantum Design Physical Property Measurement System from 1.8 to 300 K. The resistivity was measured by the standard four-probe method with the current in the ab plane. Four Au wires with diameter of 12.5 μm were spot welded to the sample. A magnetic field, up to 9 or 14 T, was applied along the c -axis, which corresponds to the magnetization easy axis [34] , [45] . Two types of pressure cells were used for this experiment. A Be-Cu/Ni-Cr-Al hybrid piston-cylinder cell, similar to the one described in ref. [46] , was used for pressures up to 2.1 GPa. A mixture of 4:6 light mineral oil: n -pentane [46] used as a pressure medium, which solidifies at ~3–4 GPa at room temperature [47] . For higher pressures, a modified Bridgman cell [48] was used to generate pressure up to 6 GPa. A 1:1 mixture of n -pentane:iso-pentane was used as a pressure medium. The solidification of this medium occurs around ~6–7 GPa at room temperature [47] , [49] . For both cells, the pressure at low temperature was determined by the superconducting transition temperature of Pb [50] measured by the resistivity. The resistivity measurement under pressure at zero field is described in ref. [16] . Data availability The data that support the findings of this study are available on request from the corresponding authors.